Full randomness from arbitrarily deterministic events Do completely unpredictable events exist? Classical physics excludes fundamental randomness. Although quantum theory makes probabilistic predictions, this does not imply that nature is random, as randomness should be certified without relying on the complete structure of the theory being used. Bell tests approach the question from this perspective. However, they require prior perfect randomness, falling into a circular reasoning. A Bell test that generates perfect random bits from bits possessing high—but less than perfect—randomness has recently been obtained. Yet, the main question remained open: does any initial randomness suffice to certify perfect randomness? Here we show that this is indeed the case. We provide a Bell test that uses arbitrarily imperfect random bits to produce bits that are, under the non-signalling principle assumption, perfectly random. This provides the first protocol attaining full randomness amplification. Our results have strong implications onto the debate of whether there exist events that are fully random. Understanding whether nature is deterministically predetermined or there are intrinsically random processes is a fundamental question that has attracted the interest of multiple thinkers, ranging from philosophers and mathematicians to physicists or neuroscientists. Nowadays, this question is also important from a practical perspective, as random bits constitute a valuable resource for applications such as cryptographic protocols, gambling or the numerical simulation of physical and biological systems. Classical physics is a deterministic theory. Perfect knowledge of the positions and velocities of a system of classical particles at a given time, as well as of their interactions, allows one to predict their future (and also past) behaviour with total certainty [1] . Thus, any randomness observed in classical systems is not intrinsic to the theory but just a manifestation of our imperfect description of the system. The advent of quantum physics put into question this deterministic viewpoint, as there exist experimental situations for which quantum theory gives predictions only in probabilistic terms, even if one has a perfect description of the preparation and interactions of the system. A possible solution to this classically counterintuitive fact was proposed in the early days of quantum physics: quantum mechanics had to be incomplete [2] and there should be a complete theory capable of providing deterministic predictions for all conceivable experiments. There would thus be no room for intrinsic randomness and any apparent randomness would again be a consequence of our lack of control over hypothetical ‘hidden variables’ not contemplated by the quantum formalism. Bell's no-go theorem [3] , however, implies that local hidden-variable theories are inconsistent with quantum mechanics. Therefore, none of these could ever render a deterministic completion to the quantum formalism. More precisely, all hidden-variable theories compatible with a local causal structure predict that any correlations among space-like separated events satisfy a series of inequalities, known as Bell inequalities. Bell inequalities, in turn, are violated by some correlations among quantum particles. This form of correlations defines the phenomenon of quantum non-locality. Now, it turns out that quantum non-locality does not necessarily imply the existence of fully unpredictable processes in nature. The reasons behind this are subtle. First of all, unpredictable processes could be certified only if the no-signalling principle holds. This states that no instantaneous communication is possible, which in turn imposes a local causal structure on events, as in Einstein's special relativity. In fact, Bohm’s theory is both deterministic and able to reproduce all quantum predictions [4] , but it is incompatible with no-signalling at the level of the hidden variables. Thus, we assume throughout the validity of the no-signalling principle. Yet, even within the no-signalling framework, it is still not possible to infer the existence of fully random processes only from the mere observation of non-local correlations. This is due to the fact that Bell tests require measurement settings chosen at random, but the actual randomness in such choices can never be certified. The extremal example is given when the settings are determined in advance. Then, any Bell violation can easily be explained in terms of deterministic models. As a matter of fact, super-deterministic models, which postulate that all phenomena in the universe, including our own mental processes, are fully predetermined, are by definition impossible to rule out. These considerations imply that the strongest result on the existence of randomness one can hope for using quantum non-locality is stated by the following possibility: given a source that produces an arbitrarily small but non-zero amount of randomness, can one still certify the existence of completely random processes? Here, we show that this is the case for a very general, and physically meaningful, set of randomness sources. This includes subsets of the well-known Santha–Vazirani sources [5] as particular cases. Besides the philosophical and physics-foundational implications, our results provide a protocol for full randomness amplification using quantum non-locality. Randomness amplification is an information-theoretic task whose goal is to use an input source of imperfectly random bits to produce perfect random bits. Santha and Vazirani [5] proved that randomness amplification is impossible using classical resources. This is in a sense intuitive, in view of the absence of any intrinsic randomness in classical physics. In the quantum regime, randomness amplification has been recently studied by Colbeck and Renner [6] . They proved how input bits with very high initial randomness can be mapped into arbitrarily pure random bits, and conjectured that randomness amplification should be possible for any initial randomness [6] . Our results also solve this conjecture, as we show that quantum non-locality can be exploited to attain full randomness amplification. Previous work Before presenting our results, it is worth commenting on previous works on randomness in connection with quantum non-locality. In the study by Pironio et al . [7] , it was shown how to bound the intrinsic randomness generated in a Bell test. These bounds can be used for device-independent randomness expansion, following a proposal by Colbeck [8] , and to achieve a quadratic expansion of the amount of random bits (see refs 9 , 10 , 11 , 12 for further works on device-independent randomness expansion). Note however that, in randomness expansion, one assumes instead, from the very beginning, the existence of an input seed of free random bits, and the main goal is to expand this into a larger sequence. The figure of merit is the ratio between the length of the final and initial strings of free random bits. Finally, other recent works have analysed how a lack of randomness in the measurement choices affects a Bell test [13] , [14] , [15] and the randomness generated in it [16] . Definition of the scenario From an information perspective, our goal is to construct a protocol for full randomness amplification based on quantum non-locality. In randomness amplification, one aims at producing arbitrarily free random bits from many uses of an input source of imperfectly random bits. A random bit b is said to be free if it is uncorrelated from any classical variables e generated outside the future light-cone of b (of course, the bit b can be arbitrarily correlated with any event inside its future light-cone). This requirement formalizes the intuition that the only systems that may share some correlation with b are the ones that are influenced by b . Note also that this definition of randomness is strictly stronger than the demand that b is uncorrelated with any classical variable generated in the past light-cone of the process. This is crucial if the variables e and b are generated by measuring on a correlated quantum system. In this case, even if both systems interacted somewhere in the past light-cone of b , the variable e is not produced until the measurement is performed, possibly outside both past and future light-cones. Furthermore, we say that a random bit is ε -free if any correlations with events outside its future light-cone are bounded by ε , as explained in what follows. Source produces a sequence of bits x 1 , x 2 ,… x j ,…, with x j =0 or 1 for all j , see Fig. 1 , which are ε -free. 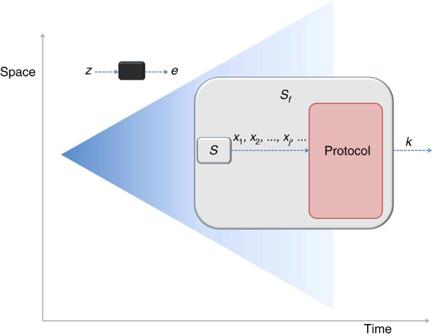Figure 1: Local causal structure and randomness amplification. A sourceproduces a sequencex1,x2,…xj,… of imperfect random bits. The goal of randomness amplification is to produce a new sourceof perfect random bits, that is, to process the initial bits so as to get a final bitkfully uncorrelated (free) from all events outside the future light cone of all the bitsxjproduced by the source. In other words,kis free if it is uncorrelated from any event outside the light cone shown in this figure. Any such event can be modelled by a measurementz, with an outcomee, on some physical system. This system may be under the control of an adversary Eve, interested in predicting the value ofk. More precisely, each bit j contains some randomness, in the sense that the probability P ( x j |all other bits, e ) that it takes a given value x j , conditioned on the values of all the other bits produced by , as well as the variable e , is such that Figure 1: Local causal structure and randomness amplification. A source produces a sequence x 1 , x 2 ,… x j ,… of imperfect random bits. The goal of randomness amplification is to produce a new source of perfect random bits, that is, to process the initial bits so as to get a final bit k fully uncorrelated (free) from all events outside the future light cone of all the bits x j produced by the source. In other words, k is free if it is uncorrelated from any event outside the light cone shown in this figure. Any such event can be modelled by a measurement z , with an outcome e , on some physical system. This system may be under the control of an adversary Eve, interested in predicting the value of k . Full size image for all j , where 0< ε ≤1/2. Given our previous definition of ε -free bits, the variable e represents events outside the future light-cone of all the x j 's. Free random bits correspond to and deterministic ones to ε =0. More precisely, when ε =0 the bound (1) is trivial and no randomness can be certified. We refer to as an ε -source, and to any bit satisfying (1) as an ε -free bit. The aim of randomness amplification is to generate, from arbitrarily many uses of , a final source of ε f -free bits with arbitrarily close to 1/2. If this is possible, no cause e can be assigned to the bits produced by , which are then fully unpredictable. Note that, in our case, we require the final bits to be fully uncorrelated from e . When studying randomness amplification, the first and most fundamental question is whether the process is at all possible. This is the question we consider and solve in this work. Thus, we are not concerned with efficiency issues, such as the rate of uses of required per final bit generated by , and, without loss of generality, restrict our analysis to the problem of generating a single final free random bit k . Our relevant figure of merit is just the quality, measured by ε f , of the final bit. Of course, efficiency issues are relevant when considering applications of randomness amplification protocols for information tasks, but this is beyond the scope of this work. The randomness amplification protocols we consider exploit quantum non-locality. This idea was introduced in the study by Colbeck and Renner [6] , where a protocol was presented in which the source is used to choose the measurement settings by two distant observers, Alice and Bob, in a Bell test [17] involving two entangled quantum particles. The measurement outcome obtained by one of the observers, say Alice, in one of the experimental runs (also chosen with ) defines the output random bit. Colbeck and Renner proved how input bits with high randomness, of 0.442< ε ≤0.5, can be mapped into arbitrarily free random bits of ε f → 1/2. In our case, the input ε -source is used to choose the measurement settings in a multipartite Bell test involving a number of observers, which depends both on the input ε and the target ε f . After verifying that the expected Bell violation is obtained, the measurement outcomes are combined to define the final bit k . For pedagogical reasons, we adopt a cryptographic perspective and assume the worst-case scenario where all the devices we use may have been prepared by an adversary Eve equipped with arbitrary non-signalling resources, possibly even supra-quantum ones. In the preparation, Eve may have also had access to and correlated the bits it produces with some physical system at her disposal, represented by a black box in Fig. 1 . Without loss of generality, we can assume that Eve can reveal the value of e at any stage of the protocol by measuring this system. Full randomness amplification is then equivalent to proving that Eve's correlations with k can be made arbitrarily small. An important comment is now in order that applies to all further discussion as well as the protocol subsequently presented. For convenience, we represent (see Figs 1 and 2 ) as a single source generating all the inputs and delivering them among the separated boxes without violating the no-signalling principle. However, this is not the scenario in practice. Operationally, each user generates his input from a local source in his lab. However, all these sources can be arbitrarily correlated to the sources of the other users with each other, without violating the bound on the correlations given by (1) and thus can be seen as a single ε -source . With this understanding, we proceed to discuss a single effective source in the rest of the text. 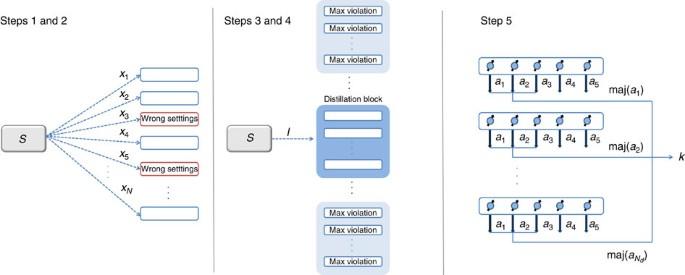Figure 2: Protocol for full randomness amplification based on quantum non-locality. In the first two steps, allNquintuplets measure their devices, where the choice of measurement is done using theε-source. Although it is illustrated here as a single source for convenience, we recall that it represents the collection of sources that each space-like separated party locally possesses with all their outputs being correlated to form anε-source. The quintuplets whose settings happen not to take place in the five-party Mermin inequality are discarded (in red). In steps 3 and 4, the remaining quintuplets are grouped into blocks. One of the blocks is chosen as the distillation block, using again, whereas the others are used to check the Bell violation. In the fifth step, the random bitkis extracted from the distillation block. Figure 2: Protocol for full randomness amplification based on quantum non-locality. In the first two steps, all N quintuplets measure their devices, where the choice of measurement is done using the ε -source . Although it is illustrated here as a single source for convenience, we recall that it represents the collection of sources that each space-like separated party locally possesses with all their outputs being correlated to form an ε -source. The quintuplets whose settings happen not to take place in the five-party Mermin inequality are discarded (in red). In steps 3 and 4, the remaining quintuplets are grouped into blocks. One of the blocks is chosen as the distillation block, using again , whereas the others are used to check the Bell violation. In the fifth step, the random bit k is extracted from the distillation block. Full size image Partial randomness from GHZ-type paradoxes Bell tests for which quantum correlations achieve the maximal non-signalling violation, also known as Greenberger–Horne–Zeilinger (GHZ)-type paradoxes [18] , are necessary for full randomness amplification. This is due to the fact that unless the maximal non-signalling violation is attained, for sufficiently small ε , Eve may fake the observed correlations with classical deterministic resources. Nevertheless, GHZ-type paradoxes are not sufficient. In fact, given any function of the measurement outcomes, it is always possible to find non-signalling correlations that (i) maximally violate the three-party GHZ paradox [18] but (ii) assign a deterministic value to that function of the measurement outcomes. This observation can be checked for all unbiased functions mapping {0,1} 3 to {0,1} (there are of those) through a linear programme analogous to the one used in the proof of the Lemma below. As a simple example, consider the particular function defined by the outcome bit of the first user. This can be fixed by using a tripartite no-signalling probability distribution consisting of a deterministic distribution for the first party and a Popescu–Rohrlich box [19] for the second and third party. However, for five parties, the latter does not hold good. Consider now any correlations attaining the maximal violation of the five-party Mermin inequality [20] . In each run of this Bell test, measurements (inputs) x =( x 1 ,…, x 5 ) on five distant black boxes generate five outcomes (outputs) a =( a 1 ,…, a 5 ), distributed according to a non-signalling conditional probability distribution P ( a | x ), see Supplementary Note 1 . Both inputs and outputs are bits, as they can take two possible values, x i , a i ε{0,1} with i =1,…,5. The inequality can be written as with coefficients where and That is, only half of all possible combinations of inputs, namely those in = 0 1 , occur in the Bell inequality. This inequality may be thought of as a non-local game in which the parties are required to minimize the parity of their outputs when the sum of their inputs is 1 or 5, whereas minimizing the inverse parity of the outputs when their inputs sum to 3. It turns out that the minimum achievable with classical strategies is 6. The maximal, non-signalling and algebraic, violation of the inequality corresponds to the situation in which the left-hand side of (2) is zero. The key property of inequality (2) is that its maximal violation can be attained by quantum correlations, and, further, one can construct a function of the outcomes that is not completely determined. Take the bit corresponding to the majority-vote function of the outcomes of any subset of three out of the five observers, say the first three. This function is equal to zero if at least two of the three bits are equal to zero and equal to one otherwise. We show that Eve's predictability on this bit is at most 3/4. We state this result in the following Lemma: Lemma: Let a five-party non-signalling conditional probability distribution P ( a | x ) in which inputs x =( x 1 ,…, x 5 ) and outputs a=( a 1 ,…, a 5 ) are bits. Consider the bit maj( a )ε{0,1} defined by the majority-vote function of any subset consisting of three of the five measurement outcomes, say the first three, a 1 , a 2 and a 3 . Then, all non-signalling correlations attaining the maximal violation of the five-party Mermin inequality are such that the probability that maj( a ) takes a given value, say 0, is bounded by Proof: This result was obtained by solving a linear programme. Therefore, the proof is numeric but exact. Formally, let P ( a|x ) be a five-partite non-signalling probability distribution. For x = x 0 ε, we performed the maximization, which yields the value P max =3/4. As the same result holds for P (maj( a )=1| x 0 ), we get the bound 1/4≤ P (maj( a )=0)≤3/4. As a further remark, note that a lower bound to P max can easily be obtained by noticing that one can construct conditional probability distributions P ( a | x ) that maximally violate five-partite Mermin inequality (2) for which at most one of the output bits (say a 1 ) is deterministically fixed to either 0 or 1. If the other two output bits ( a 2 , a 3 ) were to be completely random, the majority-vote of the three of them maj( a 1 , a 2 , a 3 ) could be guessed with a probability of 3/4. Our numerical results say that this turns out to be an optimal strategy. The previous lemma strongly suggests that, given an ε -source with any 0<ε≤1/2 and quantum five-party non-local resources, it should be possible to design a protocol to obtain an ε i -source of ε i =1/4. We do not explore this possibility here but rather use the partial unpredictability in the five-party Mermin Bell test as building block of our protocol for full randomness amplification. To complete it, we must equip it with two essential components: (i) an estimation procedure that verifies that the untrusted devices do yield the required Bell violation; and (ii) a distillation procedure that, from sufficiently many ε i -bits generated in the five-party Bell experiment, distils a single final ε f -source of ε f → 1/2. Towards these ends, we consider a more complex Bell test involving N groups of five observers (quintuplets) each. A protocol for full randomness amplification Our protocol for randomness amplification uses as resources the ε -source and 5 N quantum systems. Each of the quantum systems is abstractly modelled by a black box with binary input x and output a . The protocol processes classically the bits generated by and by the quantum boxes. When the protocol is not aborted it produces a bit k . The protocol consists of the five steps described below (see also Fig. 2 ). In step 1: is used to generate N quintuple-bits x 1 ,… x N , which constitute the inputs for the 5 N boxes and are distributed among them without violating no-signalling. The boxes then provide N output quintuple-bits a 1 ,… a N . In step 2: The quintuplets such that x ∉ are discarded. The protocol is aborted if the number of remaining quintuplets is < N /3. (Note that the constant factor 1/3 is arbitrary. In fact, it is enough to demand that the number of remaining quintuplets is larger than N / c , with c >1. See the Supplementary Note 2 ). In step 3: The quintuplets left after step 2 are organized in N b blocks each one having N d quintuplets. The number N b of blocks is chosen to be a power of 2. For the sake of simplicity, we relabel the index running over the remaining quintuplets, namely x 1 ,… X N b N d and outputs a 1 ,… a N b N d . The input and output of the j -th block are defined as y j =( X ( j − 1 ) N d + 1 ,… X ( j − 1 ) N d + N d ) and b j =( a ( j –1) N d+1 ,… a ( j –1) N d + N d ), respectively, with j ε{1,…,N b }. The random variable l ε{1,…N b } is generated by using log 2 N b further bits from . The value of l specifies that block ( b l , y l ) is chosen to generate k , that is, the distilling block. We define . The other N b –1 blocks are used to check the Bell violation. In step 4: The function tells whether block ( b , y ) features the right correlations ( r =1) or the wrong ones ( r =0), in the sense of being compatible with the maximal violation of inequality (2). This function is computed for all blocks but the distilling one. The protocol is aborted unless all the blocks give the right correlations, Note that the abort/no-abort decision is independent of whether the distilling block l is right or wrong. In step 5: If the protocol is not aborted then k is assigned a bit generated from b l =( a 1 ,… a N d ) as Here f :{0, 1} N → {0, 1} is a function whose existence is proven in the Supplementary Note 2 , whereas maj( a i )ε{0, 1} is the majority-vote among the three first bits of the quintuple string a i . At the end of the protocol, the bit k is potentially correlated with the settings of the distilling block , the bit g defined in (9), and the information In addition, an eavesdropper Eve might have access to a physical system correlated with k , which she can measure at any stage of the protocol. This system is not necessarily classical nor quantum, the only assumption about it is that measuring it does not produce instantaneous signalling anywhere else. The measurements that Eve can perform on her system are labelled by z , and the corresponding outcomes by e . In summary, after performing the protocol all the relevant information is with statistics described by an unknown conditional probability distribution . When the protocol is aborted ( g =0) there is no value for k . Therefore, to have a well-defined distribution in all cases, we set k =0 when g =0—that is , where is the Kronecker tensor. To assess the quality of our protocol for full randomness amplification, we compare it with an ideal protocol having the same marginal for the variables and the physical system described by e , z . That is, the global distribution of the ideal protocol is where is the marginal of the distribution generated by the real protocol. Note that, consistently, in the ideal distribution we also set k =0 when g =0. Our goal is that the statistics of the real protocol P is indistinguishable from the ideal statistics P ideal . We consider the optimal strategy to discriminate between P and P ideal , which obviously involves having access to all possible information and the physical system e , z . As shown in the study by Masanes [21] , the optimal probability for correctly guessing between these two distributions is Note that the second term can be understood as (one half of) the variational distance between P and P ideal generalized to the case when the distributions are conditioned on an input z . The following theorem is proven in the Supplementary Note 2 . Theorem: Let be the probability distribution of the variables generated during the protocol and the adversary's physical system e , z ; and let be the corresponding ideal distribution (11). The optimal probability of correctly guessing between the distributions P and P ideal satisfies where the real numbers α , β fulfil 0< α <1< β . Now, the right-hand side of (13) can be made arbitrary close to 1/2, for instance by setting and increasing N d subject to the condition N d N b > N /3. (Note that log 2 (1− ε )<0.) In the limit of large N d the probability P (guess) tends to 1/2, which implies that the optimal strategy is as good as tossing a coin. In this case, the performance of the protocol is indistinguishable from that of an ideal one. This is known as universally composable security and accounts for the strongest notion of cryptographic security (see refs 21 , 22 ). Let us discuss the implications and limitations of our result. Note first that step 2 in the protocol involves a possible abortion (a similar step can also be found in the study by Colbeck and Renner [6] ). Hence, only those ε -sources with a non-negligible probability of passing step 2 can be amplified by our protocol. The abortion step can be relaxed by choosing a larger value of the constant c used for rejection. Yet, in principle, it could possibly exclude some of the ε -sources defined in (1). Notice, however, that demanding that step 2 is satisfied with non-negligible probability is just a restriction on the statistics seen by the honest parties P ( x 1 ,…, x n ) and does not imply any restriction on the value of ε in ε ≤ P ( x 1 ,…, x n | e )≤(1− ε ), which can be arbitrarily small. Also, we identify at least two reasons why sources that fulfil step 2 with high probability are the most natural in the context of randomness amplification. First, from a cryptographic perspective, if the observed sequence x 1 ,…, x n does not fulfil step 2, then the honest parties will abort any protocol, regardless of whether a condition similar to step 2 is included. The reason is that such sequence would be extremely atypical in a fair source P ( x 1 ,…, x n )=1/2 n and thus the honest players will conclude that the source is intervened by a malicious party or seriously damaged. Moreover, as discussed in the Supplementary Note 3 , imposing that the source has unbiased statistics from the honest parties' point of view does not imply any restriction on Eve's predictability. Second, from a more fundamental viewpoint, the question of whether truly random events exist in nature is interesting as the observable statistics of many physical processes look random, that is, they are such that P ( x 1 ,…, x n )=1/2 n . If every process in nature was such the observable statistics does not fulfil step 2, the problem of whether truly random processes exist would hardly have been considered relevant. Finally, note that possible sources outside this subclass do not compromise the security of the protocol, only its probability of being successfully implemented. Under the conditions demanded in step 2, our protocol actually goes through for sources more general than those in (1). These are defined by the following restrictions, for any pair of functions G ( n , ε ), F ( n , ε ) defining the lower and upper bounds to Eve's control on the bias of each bit fulfilling the conditions G ( n , ε )>0 and lim n →∞ F ( n , ε )=0. In fact, this condition is sufficient for our amplification protocol to succeed, see also Supplementary Notes 2 and 3 . To complete the argument, we must mention that according to quantum mechanics, given a source that passes step 2, we can in principle implement the protocol with success probability equal to one, P ( g =1)=1. It can be immediately verified that the qubit measurements X or Y on the quantum state , with |0› and |1› the eigenstates of Z , yield correlations that maximally violate the five-partite Mermin inequality in question. (In a realistic scenario the success probability P ( g =1) might be lower than one but our theorem warrants that the protocol is still secure). We can now state the main result of our work. Full randomness amplification: a perfect free random bit can be obtained from sources of arbitrarily weak randomness using non-local quantum correlations. We would like to conclude by explaining the main intuitions behind the proof of the previous theorem. As mentioned, the protocol builds on the five-party Mermin inequality because it is the simplest GHZ paradox allowing some randomness certification. The estimation part, given by step 4, is rather standard and inspired by estimation techniques introduced in the study by Barrett et al . [23] , which were also used in the study by Colbeck and Renner [6] in the context of randomness amplification. The most subtle part is the distillation of the final bit in step 5. Naively, and leaving aside estimation issues, one could argue that it is nothing but a classical processing by means of the function f of the imperfect random bits obtained via the N d quintuplets. But this seems in contradiction with the result by Santha and Vazirani [5] proving that it is impossible to extract by classical means a perfect free random bit from imperfect ones. This intuition is, however, misleading. Indeed, the Bell certification allows applying techniques similar to those obtained in the study by Masanes [21] in the context of privacy amplification against non-signalling eavesdroppers. There it was shown how to amplify the privacy, that is the unpredictability, of one of the measurement outcomes of bipartite correlations violating a Bell inequality. The key point is that the amplification or distillation, is attained in a deterministic manner. That is, contrary to standard approaches, the privacy amplification process described in the study by Masanes [21] does not consume any randomness. Clearly, these deterministic techniques are extremely convenient for our randomness amplification scenario. In fact, the distillation part in our protocol can be seen as the translation of the privacy amplification techniques of Masanes [21] to our more complex scenario, involving now five-party non-local correlations and a function of three of the measurement outcomes. To summarize, we have presented a protocol that, using quantum non-local resources, attains full randomness amplification, a task known to be impossible classically. As our goal was to prove full randomness amplification, our analysis focuses on the noise-free case. In fact, the noisy case only makes sense if one does not aim at perfect random bits and bounds the amount of randomness in the final bit. Then, it should be possible to adapt our protocol to get a bound on the noise it tolerates. Other open questions that our results offer as challenges consist of extending randomness amplification to other randomness sources, studying randomness amplification against quantum eavesdroppers or the search of protocols in the bipartite scenario. From a more fundamental perspective, our results imply that there exist experiments whose outcomes are fully unpredictable. The only two assumptions for this conclusion are the existence of events with an arbitrarily small but non-zero amount of randomness that pass step 2 of our protocol and the validity of the no-signalling principle. Dropping the first assumption would lead to super-determinism or to accept that the only source of randomness in nature is one that does not pass step 2 of our protocol, and in particular, one that does not look unbiased. On the other hand, dropping the second assumption would imply abandoning a local causal structure for events in space-time. However, this is one of the most fundamental notions of special relativity. How to cite this article: Gallego, R. et al . Full randomness from arbitrarily deterministic events. Nat. Commun. 4:2654 doi: 10.1038/ncomms3654 (2013).